Structure of a photosynthetic reaction centre determined by serial femtosecond crystallography Serial femtosecond crystallography is an X-ray free-electron-laser-based method with considerable potential to have an impact on challenging problems in structural biology. Here we present X-ray diffraction data recorded from microcrystals of the Blastochloris viridis photosynthetic reaction centre to 2.8 Å resolution and determine its serial femtosecond crystallography structure to 3.5 Å resolution. Although every microcrystal is exposed to a dose of 33 MGy, no signs of X-ray-induced radiation damage are visible in this integral membrane protein structure. X-ray crystallography is the most successful method for determining new membrane protein structures. Membrane protein crystallization, however, continues to pose many challenges because of the inherent conflict between hydrophilic and hydrophobic domains within the protein, flexible loops and low protein expression yields [1] . When crystals are obtained they are often small, frequently diffract to low resolution, and crystal collection and cryoprotection can introduce additional challenges. As such, it has become increasingly common to use synchrotron-based microfocus beamlines [2] to screen large numbers of very small membrane protein crystals and to merge diffraction data from multiple crystals so as to recover complete diffraction data. Serial femtosecond crystallography (SFX) brings a new dimension to the challenge of screening small crystals. This approach has been developed as a high-resolution structural method [3] , [4] , [5] , [6] at X-ray free-electron lasers (XFELs) and allows diffraction data to be collected at room temperature from thousands of randomly oriented, fully hydrated micron-sized crystals injected into the XFEL beam using a microjet [7] , [8] . In combination with rapid X-ray detectors [9] , it is possible to collect millions of frames in a 12 hour shift at the Linac Coherent Light Source (LCLS) [10] , which provides extremely intense X-ray pulses at a repetition rate of 120 Hz. In addition to microfocusing, the key advantage of XFEL-based serial femtosecond crystallography over conventional diffraction strategies using synchrotron radiation is that each XFEL pulse of ∼ 10 12 X-ray photons is only a few tens of femtoseconds in duration. This allows diffraction data to be recorded using brilliant X-ray bursts before the microcrystals have time to be destroyed by the effects of radiation damage [11] , [12] , [13] . The first proof-of-principle SFX structures were of photosynthetic membrane protein complexes [3] , [4] up to 8.2 Å resolution and were recovered from diffraction data recorded at the atomic, molecular and optical science experimental station [14] of the LCLS [10] using the CAMP instrument [15] . High-resolution SFX structures of the soluble proteins lysozyme [5] and cathepsin B [6] (1.9 and 2.1 Å resolution, respectively) were reported following the commissioning of the coherent X-ray imaging (CXI) instrument [16] , which operates at shorter wavelengths. Despite these advances, diffraction data recorded at the LCLS from membrane protein microcrystals have been considerably weaker than data recorded from microcrystals of soluble proteins. The highest-resolution membrane protein SFX structure reported to date is from photosystem II (ref. 17 ) and extends only to 5.7 Å resolution, a resolution at which side chains cannot usually be resolved. In this work, microcrystals of the photosynthetic reaction centre from Blastochloris viridis (RC vir ), a four-subunit integral membrane protein complex of 135 kDa, are grown in a lipidic sponge phase (LSP) [4] and exposed to the focused XFEL beam of the LCLS [10] . Diffraction data from 1,175 crystals are merged to recover a SFX structure to 3.5 Å resolution. Although the X-ray exposure for each and every microcrystal is 33 MGy, which is approximately two orders of magnitude beyond that normally suitable for room temperature data collection, no signs of radiation damage are visible in the resulting electron density. These results demonstrate the considerable potential of XFEL-based SFX when applied to the challenging field of membrane protein structural biology. Diffraction data and electron density maps Microcrystals of RC vir were grown in a LSP [4] and transported at room temperature to the LCLS. LSP crystallization [18] , [19] is a liquid analogue of the lipidic cubic phase crystallization [19] , [20] , [21] , which aids membrane protein crystal growth by forming a continuous lipidic bilayer mimicking the natural membrane environment. The LSP-grown RC vir microcrystals were injected as a microjet [7] , [8] across the focused XFEL beam of the LCLS and diffraction data to 2.8 Å resolution ( Fig. 1 ) were collected on a Cornell-SLAC Pixel Array detector [9] at the CXI instrument [16] . As this beamline operates at a short wavelength ( ∼ 1.4 Å), it was possible to extend our earlier 8.2 Å resolution RC vir SFX structure [4] to 3.5 Å resolution, at which most side chains can be assigned without ambiguity. 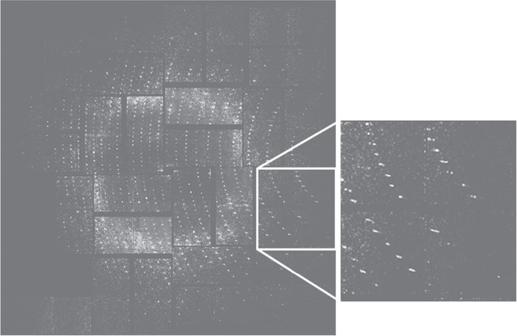Figure 1: SFX diffraction data. Data were recorded on the Cornell-SLAC Pixel Array detector from microcrystals of RCvirat the CXI beamline of the LCLS. The resolution limit at the edge of the detector was 2.62 Å. Diffractions spots were observed up to 2.8 Å resolution. Figure 1: SFX diffraction data. Data were recorded on the Cornell-SLAC Pixel Array detector from microcrystals of RC vir at the CXI beamline of the LCLS. The resolution limit at the edge of the detector was 2.62 Å. Diffractions spots were observed up to 2.8 Å resolution. Full size image From two million images recorded during 5 h of beamtime, 3% were identified as containing more than ten spots using the software Cheetah [22] , of which 5,767 showed diffraction when examined visually. Indexing was performed using the CrystFEL suite [23] and resulted in 1,175 processed diffraction images, which were scaled and merged using Monte Carlo methods [24] . Diffraction data were cut at 3.5 Å resolution for which I / σ ≥2 and the completeness ≥92% ( Supplementary Fig. S1 , Table 1 and Supplementary Table S1 ). The RC vir structure was solved by molecular replacement, yielding the same crystal packing (space group P2 1 2 1 2 1 ; a =57.9 Å, b =84.8 Å, c =384.3 Å) as previously reported [4] . This is compared with the crystal packing of other RC vir structures in Supplementary Table S2 . Table 1 Data collection and refinement statistics. 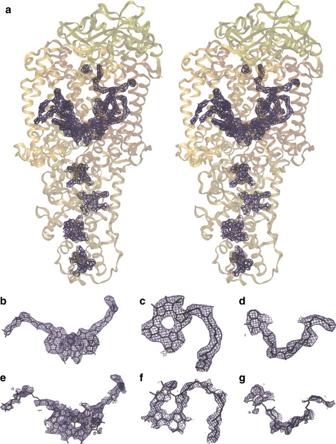Figure 2:Electron density maps calculated from the SFX RCvirdiffraction data. (a) Stereo view of the 2mFobs−DFcalcelectron density map for the RCvircofactors. Close-up views of the 2mFobs−DFcalcelectron density map are shown for (b) the special pair, (c) the L-branch bacteriopheophytin and (d) the menaquinone in theQApocket. Close-up views of the composite omit electron density map are shown for (e) the special pair, (f) the L-branch bacteriopheophytin and (g) the menaquinone. The composite omit map, which suffers from less model bias than the 2mFobs−DFcalcelectron density map, better illustrates the quality of the SFX diffraction data. All panels are contoured at 1.0σ. Full size table Figure 2a shows the 2mF obs −DF calc electron density map in stereo contoured around all cofactors after structural refinement to 3.5 Å resolution, for which R -factor and R free values of 29.4 and 32.7% were recovered. A closer view of this electron density illustrates that the bacteriochlorophyll tails of the special pair are unbroken ( Fig. 2b ); that the bacteriopheophytin cofactors do not have a metal centre ( Fig. 2c ); and that the menaquinone head group and tail are resolved within the Q A pocket ( Fig. 2d ). Similarly, the electron density recovered when calculating the composite omit map ( Fig. 2e–g ), which displays less model bias than the 2mF obs −DF calc map, also reveals clear electron density for these cofactors. As key quality indicators such as I / σ , CC 1/2 , completeness and R free vary smoothly as the resolution is extended ( Supplementary Fig. S1 ), our choice of cutting the data to 3.5 Å resolution might be viewed as unnecessarily conservative. Calculation of the composite omit map at 3.3 Å resolution ( Supplementary Fig. S2 ), however, does not reveal new details within the map and the electron density for the cofactors appears more broken than when the data are cut at 3.5 Å resolution. Figure 2: Electron density maps calculated from the SFX RC vir diffraction data. ( a ) Stereo view of the 2mF obs −DF calc electron density map for the RC vir cofactors. Close-up views of the 2mF obs −DF calc electron density map are shown for ( b ) the special pair, ( c ) the L-branch bacteriopheophytin and ( d ) the menaquinone in the Q A pocket. Close-up views of the composite omit electron density map are shown for ( e ) the special pair, ( f ) the L-branch bacteriopheophytin and ( g ) the menaquinone. The composite omit map, which suffers from less model bias than the 2mF obs −DF calc electron density map, better illustrates the quality of the SFX diffraction data. All panels are contoured at 1.0 σ . Full size image The quality of the electron density maps at 3.5 Å resolution is striking given that the overall multiplicity is 27 ( Table 1 ) and is orders of magnitude lower than that reported for high-resolution SFX structures of lysozyme [5] (379) and cathepsin B [6] (7,808); there is considerable variation in the crystallographic observations that are averaged to recover I hkl for each and every hkl value [24] ( Supplementary Fig. S3 illustrates sets of observations for representative hkl values); and data processing with a long axis ( c =384.3 Å) introduces experimental challenges due to the close spacing of diffraction spots in reciprocal space. As a result, the correlation coefficient of the SFX data when split into two halves is lower when projected along the c axis relative to that recovered when projecting along the a or b axes ( Supplementary Fig. S1a,b ). These findings indicate the power of SFX multicrystal averaging to recover high-multiplicity data sets for which the electron density maps are better than normally expected using traditional quality indicators developed for single crystal data sets. Radiation damage A groundbreaking aspect of XFEL-based SFX is that the use of ultrafast X-ray pulses enables the traditional radiation damage barrier of structural biology [25] to be side-stepped [11] , [12] . In this work, each microcrystal was exposed to a 42-fs X-ray pulse of 4 × 10 11 9.34 keV photons focused into a spot of 10 μm 2 . This corresponds to a dose of 33 MGy deposited into each and every microcrystal (calculated using RADDOSE [26] ), which equates to instantaneously depositing the heat output of a 1-kW kettle running for 9 h into 1 litre of water (1 MGy=1 MJ absorbed by 1 kg of matter). This dose is approximately two orders of magnitude above that normally acceptable for traditional room-temperature crystallography and is equal to an empirical X-ray dose limit found at cryogenic temperatures [25] . Under these conditions, approximately four primary photo-ionization events occur within every RC vir molecule, which in turn induce a further 200 secondary ionization events [27] . As with studies of lysozyme under similar experimental conditions [5] , the RC vir electron density appears unaffected by these damaging events. First and foremost, the SFX crystal structure of RC vir is very similar to an earlier room-temperature Laue diffraction structure [28] (pdb entry 2X5U) having a root mean squared deviation (r.m.s.d.) of 0.49 Å calculated over all C α atoms when both RC vir models are aligned on the 11 transmembrane (TM) α-helices. All C α changes have a statistical significance ≤2.0 σ and the largest changes (error-weighted difference ≥1.0 σ relative to at least 20 other C α atoms) are associated with the C- and H-subunits ( Fig. 3a ), as illustrated by calculation of the error-weighted change in internal distance matrix [29] ( Supplementary Fig. S4 ). These differences correspond to an r.m.s.d. shift of 0.71 Å for the C subunit and 0.48 Å for the H-subunit when aligned on the RC vir TM regions ( Supplementary Table S3 ). Although the crystal packing of both microcrystal and macrocrystal (that is, normal-sized crystals typically 0.2 × 0.2 × 0.5 mm 3 ) forms are similar, with both forming stacked layers of two-dimensional membrane crystals, there are differences between the protein:protein crystal packing interactions that are largely mediated by the C- and H-subunits ( Fig. 3b,c ), and these presumably underlie this structural perturbation. 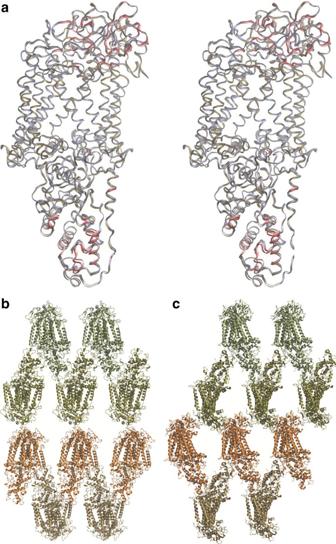Figure 3:Comparison of the RCvirSFX structure with an earlier structure. (a) Superposition in stereo of the SFX crystal structure (brown) upon the Laue diffraction RCvirstructure (white, pdb entry 2X5U). Both structures were aligned on their 11 TM helices. Regions for which the coordinate changes are ≥1.0σ(calculated according to ref.29,Supplementary Fig. S4) are marked in red and correspond to subtle backbone differences in subunits C and H. (b) Crystal packing of the LSP microcrystal form used in this SFX study. (c) Crystal packing of the LSP macrocrystal form (that is, larger crystals) used in other studies28,30. Crystal contacts differ between the microcrystal (space group P212121;a=57.9 Å;b=84.8 Å;c=384.3 Å) and macrocrystal (space group P21212;a=85 Å;b=139 Å;c=178 Å) forms. Figure 3: Comparison of the RC vir SFX structure with an earlier structure. ( a ) Superposition in stereo of the SFX crystal structure (brown) upon the Laue diffraction RC vir structure (white, pdb entry 2X5U). Both structures were aligned on their 11 TM helices. Regions for which the coordinate changes are ≥1.0 σ (calculated according to ref. 29 , Supplementary Fig. S4 ) are marked in red and correspond to subtle backbone differences in subunits C and H. ( b ) Crystal packing of the LSP microcrystal form used in this SFX study. ( c ) Crystal packing of the LSP macrocrystal form (that is, larger crystals) used in other studies [28] , [30] . Crystal contacts differ between the microcrystal (space group P2 1 2 1 2 1 ; a =57.9 Å; b =84.8 Å; c =384.3 Å) and macrocrystal (space group P2 1 2 1 2; a =85 Å; b =139 Å; c =178 Å) forms. Full size image Calculation of the mF obs −DF calc omit electron density map ( Fig. 4 ) with all Fe and Mg atoms removed from the model shows that all metal centres, which have higher photo-ionization cross-sections than other atoms in the sample, emerge as strong positive residual density peaks. The average significance of the residual mF obs −DF calc omit map peaks for the Mg atoms was 3.0 σ , whereas that for the Fe atoms was 6.0 σ , corresponding to a ratio for Mg:Fe of 50% and in agreement with that recovered (48%) using synchrotron diffraction data to 1.9 Å resolution [30] (pdb entry 2WJN). Furthermore, the 2mF obs −DF calc electron density for the residues that ligate the bacteriochlorophyll and haem metal centres is well ordered ( Fig. 4 ). 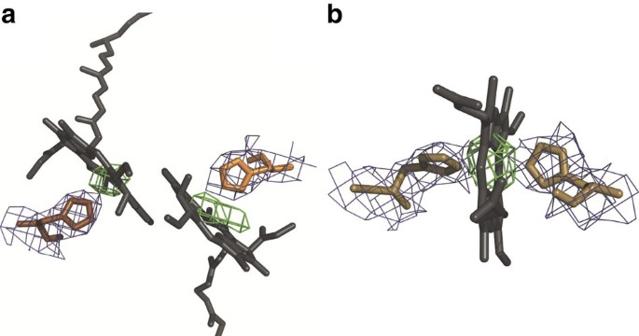Figure 4: Electron density for the metal containing cofactors. (a) mFobs−DFcalcresidual electron density (green, contoured at 1.5σ) calculated with the two Mg atoms removed from the special pair. (b) mFobs−DFcalcresidual electron density (green, contoured at 3.0σ) calculated with the Fe atom removed from haem 4. The 2mFobs−DFcalcelectron density map (blue, contoured at 1.0σ) shows the electron density for the histidine side chains coordinating (a) the Mg atoms and (b) the iron. Figure 4: Electron density for the metal containing cofactors. ( a ) mF obs −DF calc residual electron density (green, contoured at 1.5 σ ) calculated with the two Mg atoms removed from the special pair. ( b ) mF obs −DF calc residual electron density (green, contoured at 3.0 σ ) calculated with the Fe atom removed from haem 4. The 2mF obs −DF calc electron density map (blue, contoured at 1.0 σ ) shows the electron density for the histidine side chains coordinating ( a ) the Mg atoms and ( b ) the iron. Full size image Radiation damage studies of RC vir at cryogenic temperatures have identified that the covalent thioether bond linking the N-terminal cysteine residue of the tetrahaem cytochrome c subunit (CysC1) to a diacylglycerol molecule is susceptible to X-ray-induced damage. Specifically, a comparison of the electron density recovered from monochromatic data collected at 100 K using an X-ray dose of 4.4 MGy ( Fig. 5a , pdb entry 2WJM [30] ) with that recovered using a dose of 77 MGy at 100 K ( Fig. 5b , pdb entry 2WJN [30] ) reveals that this bond is completely cleaved at high dose. As the RC vir SFX diffraction data were collected at room temperature, it might be anticipated that these data would be more prone to radiation-induced damage than data collected at cryogenic temperatures. Nevertheless, the 2mF obs −DF calc SFX electron density map, calculated using a dose of 33 MGy per microcrystal, reveals continuous electron density for this bond ( Fig. 5c ). This finding clearly demonstrates that according to this internal radiation damage marker, there are no observable effects of radiation damage on the SFX crystal structure of RC vir . 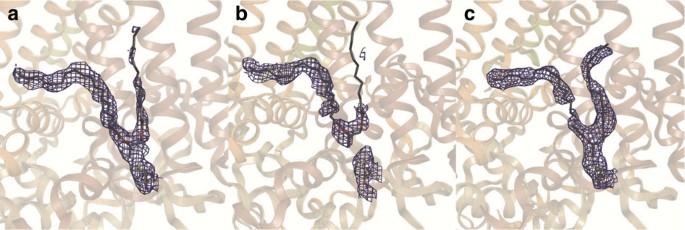Figure 5: X-ray damage to a radiation-sensitive bond. (a) Electron density illustrating the thioether covalent bond linking the N-terminal cysteine of the C subunit to a diacylglycerol molecule calculated from monochromatic diffraction data30collected at cryogenic temperatures using an X-ray dose of 4.4 MGy. (b) Electron density calculated when the X-ray dose at cryogenic temperatures was 77 MGy. (c) Electron density calculated from the room-temperature SFX diffraction data using an X-ray dose of 33 MGy. The continuous electron density inais highly disrupted inb, illustrating how radiation damage cleaves this covalent thioether bond. In the room temperature SFX structurec, this bond appears unaffected by radiation damage. All panels are contoured at 0.7σ. Figure 5: X-ray damage to a radiation-sensitive bond. ( a ) Electron density illustrating the thioether covalent bond linking the N-terminal cysteine of the C subunit to a diacylglycerol molecule calculated from monochromatic diffraction data [30] collected at cryogenic temperatures using an X-ray dose of 4.4 MGy. ( b ) Electron density calculated when the X-ray dose at cryogenic temperatures was 77 MGy. ( c ) Electron density calculated from the room-temperature SFX diffraction data using an X-ray dose of 33 MGy. The continuous electron density in a is highly disrupted in b , illustrating how radiation damage cleaves this covalent thioether bond. In the room temperature SFX structure c , this bond appears unaffected by radiation damage. All panels are contoured at 0.7 σ . Full size image XFELs, by providing extremely brilliant X-ray pulses of femtoseconds in duration, have the potential to have major impact on the field of structural biology. Earlier proof-of-principle studies demonstrated that SFX is a high-resolution method when studying microcrystals of soluble proteins [5] , [6] . From a long-term perspective, the impact of XFEL-based SFX on structural biology will depend on its ability to address problems that are challenging or intractable using traditional data collection strategies at synchrotron radiation sources. Membrane protein crystallography remains a major challenge for the structural biology community [1] . Our results establish that SFX structures can be recovered from LSP membrane protein microcrystals to a resolution where protein side chains, cofactors and bound lipid molecules can be unambiguously resolved. Moreover, no indications of radiation-induced damage are visible in radiation-sensitive covalent bonds or metal cofactors. These findings provide a platform from which future challenges in membrane protein structural biology can be addressed with confidence. Purification and LSP batch crystallization The photosynthetic reaction centre from Bl. viridis was purified [4] using 250 ml POROS ‘50 micron’ HQ media (Applied Biosystems Europe BV) packed in an XK 50/20 column (GE Healthcare) equilibrated with 20 mM Tris-HCl, pH 8.5, and 1% lauryldimethylamine-oxide (LDAO). The protein was eluted using a linear gradient of 0–0.5 M NaCl in 20 mM Tris-HCl, pH 8.5, and 1% LDAO, and subsequently loaded onto a HiPrep 26/60 Sephacryl S-300 column (GE Healthcare) equilibrated with 10 mM Tris-HCl, pH 8.5, and 0.1% LDAO. This protocol yielded ∼ 3 mg of pure RC vir per litre of cell culture. Batch crystallization trials were prepared in septum-sealed glass vials (Sigma-Aldrich) containing 100 μl protein (25–35 mg ml −1 ), 100 μl LSP (12% monoolein, 17.5% Jeffamine M-600, 1.0 M Hepes (pH 8.0), 0.7 M (NH 4 ) 2 SO 4 and 2.5% 1,2,3-heptanetriol) and 100 μl of 1.0–1.2 M trisodium citrate. The setups were left to equilibrate for 2–4 weeks at 20 °C and were shipped at room temperature to the LCLS. Sample injection and data collection RC vir crystals were delivered to the injector nozzle via a syringe [31] and were injected into the XFEL beam at a flow rate of 10 μl min −1 . The liquid capillary of the nozzle had an inner diameter of 100 μm and the liquid was focused by helium gas to a continuous jet stream of ∼ 4 μm in diameter. The X-rays were aligned so as to hit the liquid in the jet region before the Rayleigh breakup of the jet into droplets. All microcrystals were filtered through a 20-μm cutoff filter (VICI AG International) before injection. Diffraction data were collected at the CXI [16] beamline at the LCLS in January 2011. Diffraction data were recorded on Cornell-SLAC Pixel Array detectors [9] , consisting of 64 tiles (each 192 pixels by 185 pixels) with a pixel size of 110 × 110 μm 2 . The X-ray wavelength at CXI was 1.32 Å, pulse energy 9.34 keV and pulse duration 42 fs. The XFEL beam was focused to a 10-μm 2 area spot and the detector distance was 142 mm from the microjet. Data processing Data were processed using the software suite CrystFEL [23] . Data from 1,175 diffraction images were indexed using an orthorhombic unit cell with unit cell axes a =57.9 Å, b =84.8 Å, c =384.3 Å and α = β = γ =90°. As every diffraction image is a still, there are no fully recorded reflections. Scaling and merging of data were thus performed using Monte Carlo methods developed by Kirian et al. [24] In parallel, scaling and merging was also performed by the CCP4 programme Aimless [32] , using the unmerged observations derived by CrystFEL. The same set of unmerged observations was sorted and grouped according to image number or unique hkl indices using the cctbx libraries [33] . Data collection statistics are summarized in Table 1 and Supplementary Table S1 , and the multiplicity of 27 is consistent across all shells. When data were split into two equal sets (consisting of even and odd images) and processed in parallel, an R split value of 37% (53% outer shell) and an internal correlation coefficient (CC 1/2 ) of 0.54 (0.32 outer shell) were recovered when merging the two halves of the data. Errors associated with indexing and integrating data along the long c axis contribute to this relatively low value of CC 1/2 ( Supplementary Fig. S1a,b ). The value of R split is consistent with distributions calculated from subsets of lysozyme data assuming a multiplicity of 27 (Supplementary Fig. S5 of ref. 5 ). Structure determination For structural analysis, diffraction data were cut at 3.5 Å resolution. PhaserMR 2.5.0 (ref. 34 ) was used to obtain a molecular replacement solution in the space group P2 1 2 1 2 1 with a search model based on the high-resolution structure of RC vir (PDB entry 2WJN). The best solutions had a translation function Z score of 32.8, a rotation function Z score of 28.6 and a log likelihood gain of 2,879. The SFX RC vir structure was refined using the CCP4 suite. Rigid body refinement was performed using 20 cycles with cofactors omitted, followed by an identical round of refinement but with all cofactors present. Jelly body refinement was used together with several rounds of Translation/Libration/Screw (TLS) refinement, converging to R work / R free =0.294/0.327 (figure of merit 0.78). During refinement, we used simple Wilson scaling and a constant density (using default values) was assigned to the region of the unit cell not occupied by protein atoms. We calculated the solvent mask using default parameters: increase van der Waals radius of non-ion atoms by 1.2 Å, increase ionic radius of potential ions by 0.8 Å and shrink the area of the mask by 0.8 Å after the calculation. Crystallographic data and refinement statistics are summarized in Table 1 . The geometry was evaluated using the MOLPROBITY [35] and PROCHECK [36] yielding 97% in the Ramachandran-favoured region and 3% in the allowed region. mF obs −DF calc omit electron density maps ( Fig. 4 ) were calculated by first removing Mg and Fe atoms from the model and then recalculating the map. Composite omit maps were calculated by Phenix [37] , using default parameters (no simulated annealing). All composite omit maps were contoured at 1 σ . Analysis of conformational differences The refined SFX structure was compared with other crystallographic structures using an error-weighted internal distance matrix analysis [29] , which builds upon the Cruickshank diffraction precision index [38] . For r.m.s.d. comparisons ( Supplementary Table S3 ), RC vir structures were first overlaid on their 11 TM helices and the r.m.s.d. calculated on C α atoms. PDB Accession code : Coordinates and structure factors for the RC vir SFX structure have been deposited in the RCSB Protein Data Bank under accession code 4CAS . How to cite this article: Johansson, L. C. et al. Structure of a photosynthetic reaction centre determined by serial femtosecond crystallography. Nat. Commun. 4:2911 doi: 10.1038/ncomms3911 (2013).